A unified strategy for the synthesis of highly oxygenated diaryl ethers featured in ellagitannins Ellagitannins are a family of polyphenols containing more than 1,000 natural products. Nearly 40% of these compounds contain a highly oxygenated diaryl ether that is one of the most critical elements to their structural diversity. Here, we report a unified strategy for the synthesis of highly oxygenated diaryl ethers featured in ellagitannins. The strategy involves oxa-Michael addition of phenols to an orthoquinone building block, with subsequent elimination and reductive aromatization. The design of the building block—a halogenated orthoquinone monoketal of gallal—reduces the usual instability of orthoquinone and controls addition/elimination. Reductive aromatization is achieved with perfect chemoselectivity in the presence of other reducible functional groups. This strategy enables the synthesis of different diaryl ethers. The first total synthesis of a natural ellagitannin bearing a diaryl ethers is performed to demonstrate that the strategy increases the number of synthetically available ellagitannins. The structural diversity of natural products often derives from the oligomerization of monomers that are specific to each family of compounds. Snyder and co-workers have divided a large number of oligomeric natural products into two categories [1] : serially and non-serially produced oligomers. In serially produced oligomers, monomers unite regiospecifically with definite bonding patterns; examples include DNA ( Supplementary Note ) and proteins. In contrast, in non-serially produced cases, oligomerization apparently unites monomers in a random manner, with no fixed position. This division can also be applied to polyphenols, although their structural diversity is sufficiently large to classify them into several structural families [2] . Polyphenols have potential applications in medicine and health enhancement. However, their structure-activity/affinity relationships are not well understood due to the difficulty in obtaining a complete collection of systematically related analogues from nature. This difficulty might be resolved through chemical synthesis if all compounds of a polyphenol family could be synthesized. The methodologies required to achieve this exhaustive synthesis would differ from those used for a one-off total synthesis of a single compound. For the exhaustive synthesis of serially produced oligomers, the procurement of all component parts and the development of effective methods for assembling the parts are the most important tasks. For exhaustive synthesis of non-serially produced oligomers, the discovery of latent systems that exhibit structural diversity and the development of methodologies to address multipoint random oligomerizations are required. Attempts to satisfy these requirements for both serially and non-serially produced polyphenols have already begun, as evidenced by the work of Ohmori et al. [3] and Snyder et al. [4] , who have developed methods for synthesizing higher catechin oligomers and programmable resveratrol oligomers, respectively. The family of ellagitannins, which consists of bioactivity- and structure-rich polyphenols [5] , [6] , has been found to contain more than 1,000 natural products to date [7] . The most basic ellagitannins consist of a glucose core with esterified galloyl and hexahydroxydiphenoyl (HHDP) groups ( Fig. 1 ); however, the simple combination of these basic constituents is insufficient to generate structural diversity. Despite Snyder's classification of ellagitannins as serially produced oligomers [1] , the reality is not that simple. The HHDP groups on the glucose cores do not appear at fixed positions. Furthermore, disorders of the routine patterns in uniting the component parts frequently appear in higher ellagitannins. In addition, the family includes numerous component parts, including overoxidation [8] , [9] , modifications of the HHDP group [10] , conjugation with other natural constituents [11] , [12] , [13] and production of the highly oxygenated diaryl ethers. Among these factors conferring structural diversity, the production of highly oxygenated diaryl ethers, C–O digallates, is the most significant. C–O digallates are structures that contain dimerized galloyl group(s) connected by a C–O bond, such as the dehydrodigalloyl (DHDG), tergalloyl and valoneoyl groups. These motifs allow oligomerization of basic ellagitannins, which expands diversity [14] . Nearly 40% of characterized natural ellagitannins contain C–O digallates. 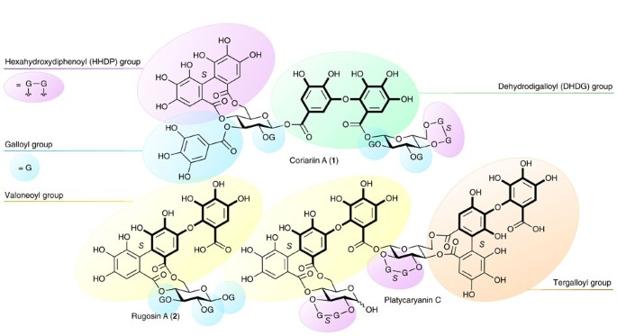Figure 1: Natural ellagitannins possessing highly oxygenated diaryl ethers. The parts indicated with bold lines are the highly oxygenated diaryl ethers, C–O digallates. Each common name is also indicated. The C–O digallates allow oligomerization of basic ellagitannins, which is a major factor in conferring structural diversity. However, the methods for synthesizing C–O digallates have been quite limited to date. Figure 1: Natural ellagitannins possessing highly oxygenated diaryl ethers. The parts indicated with bold lines are the highly oxygenated diaryl ethers, C–O digallates. Each common name is also indicated. The C–O digallates allow oligomerization of basic ellagitannins, which is a major factor in conferring structural diversity. However, the methods for synthesizing C–O digallates have been quite limited to date. Full size image For the exhaustive synthesis of ellagitannins, one of the most fundamental tasks is the formation of the chiral HHDP group, a C–C digallate, which has been achieved through several procedures [15] , [16] , [17] , [18] . The second and most impactful task would be the establishment of a methodology for synthesizing C–O digallates because their structure is the primary cause of structural diversity in this family. Therefore, establishment of this methodology should increase the number of synthetically available ellagitannins in an innovative manner. However, few reports of the synthesis of C–O digallates have appeared in the literature. One of the rare examples is Feldman’s synthesis of DHDG derivative 3 ( Fig. 2a ) [19] , [20] , [21] . This synthesis is a four-step sequence that starts from orthoquinone 4 through (1) the self-hetero Diels-Alder cycloaddition of 4 to produce a mixture of regioisomers 5a and 5b , (2) β-elimination, as indicated by the curved arrows, (3) reduction of the orthoquinone, and (4) benzylation accompanying the Smiles rearrangement [22] , which converges the mixture into 3 . Utilizing the DHDG derivative of 3 , they achieved the total synthesis of coriariin A ( 1 ) [20] , which is the sole ellagitannin containing the C–O digallate synthesized to date. However, the application of this method to HHDP-containing C–O digallates is quite difficult because the first step, the C–O bond-forming reaction, relies on the self-dimerization of 4 . 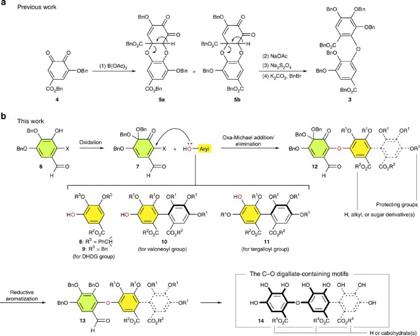Figure 2: Outlines of previous and present methods for the synthesis of C–O digallates. (a) Feldman's synthesis of the DHDG group, which was formerly the sole method for synthesizing a C–O digallate, the DHDG group, as applied to the total synthesis of ellagitannins. (b) The unified strategy of C–O digallates (this work). Oxa-Michael addition of phenols8–11to key building block7and subsequent elimination formed the C–O bond of the digallates. The design of building block7was critical. The monoketal and halogen X stabilized the structure. Halogen X made the oxa-Michael addition irreversible because leaving group X caused smooth elimination after the oxa-Michael addition. In addition, X limited the electrophilic position in oxa-Michael addition to the β-carbon of the aldehyde but not to that of the ketone. The reductive aromatization of12required selective reduction of the orthoquinone monoketal in the presence of an aldehyde, an ester in the ‘Aryl’ part, and a benzylidene acetal when8was employed. The (S)-axial chiralities of10and11are drawn tentatively; thus, usage of the corresponding (R)-isomers and the racemates is also possible. Ac, acetyl; Bn, benzyl; Ph, phenyl. Figure 2: Outlines of previous and present methods for the synthesis of C–O digallates. ( a ) Feldman's synthesis of the DHDG group, which was formerly the sole method for synthesizing a C–O digallate, the DHDG group, as applied to the total synthesis of ellagitannins. ( b ) The unified strategy of C–O digallates (this work). Oxa-Michael addition of phenols 8 – 11 to key building block 7 and subsequent elimination formed the C–O bond of the digallates. The design of building block 7 was critical. The monoketal and halogen X stabilized the structure. Halogen X made the oxa-Michael addition irreversible because leaving group X caused smooth elimination after the oxa-Michael addition. In addition, X limited the electrophilic position in oxa-Michael addition to the β-carbon of the aldehyde but not to that of the ketone. The reductive aromatization of 12 required selective reduction of the orthoquinone monoketal in the presence of an aldehyde, an ester in the ‘Aryl’ part, and a benzylidene acetal when 8 was employed. The ( S )-axial chiralities of 10 and 11 are drawn tentatively; thus, usage of the corresponding ( R )-isomers and the racemates is also possible. Ac, acetyl; Bn, benzyl; Ph, phenyl. Full size image Alternatively, Ullmann coupling can be used to prepare C–O digallates. Nishioka and co-workers [23] and Abe et al. [24] , [25] independently synthesized C–O digallates through Ullmann coupling as fully O-methylated variants. However, total synthesis via fully O-methylated ellagitannins might be unproductive because complete cleavage of methyl ethers without degradation of the other part of the molecule has been difficult. Feldman et al. [15] stated that per-O-methyl ethers are not likely to be ultimately useful in natural product synthesis. Actually, no route has resulted in unprotected ellagitannins through the methyl (Me)-protection of phenols [25] , [26] , [27] , [28] . Nonetheless, the Ullmann coupling of gallates protected by benzyl ethers, whose cleavage through hydrogenolysis is easy, is not very efficient at present [29] . In this study, we developed an entirely novel and unified strategy for the synthesis C–O digallates, including the DHDG, tergalloyl and valoneoyl groups, which is a significant step toward the exhaustive synthesis of ellagitannins. To demonstrate the effectiveness of this strategy, we performed the first total synthesis of the valoneoyl-group-containing ellagitannin rugosin A ( 2 ). Strategy Our strategy is outlined in Fig. 2b . The carboxylic acid moieties of C–O digallate-containing motifs 14 are often unequally modified with or without carbohydrates or possess differently substituted carbohydrates. Therefore, the carboxylic acid moieties must be distinguished during synthesis. To achieve this distinction, we added an aldehyde group to key synthetic intermediate 13 . The aryl–O–aryl bonds in the DHDG and valoneoyl groups are tri- ortho substituted, and their formation through cross-coupling catalysed by transition metals has been difficult [30] , [31] . Furthermore, the bond in the tergalloyl group is tetra- ortho substituted. For construction of multi-ortho-substituted aryl–O–aryl bonds, nucleophilic aromatic substitution (S N Ar) has been effective [29] , [30] . However, the reaction position of the galloyl group is electron rich, which is unfavourable to the S N Ar reaction. In this context, we planned to change the phenol to an electron-poor alkene through oxidative dearomatization. Thus, we constructed the sterically crowded aryl–O–aryl bond of 13 through oxa-Michael addition of a phenolic hydroxy group of 8 (ref. 32 ), 9 (ref. 33 ), 10 and 11 for the DHDG, valoneoyl, and tergalloyl groups to orthoquinone monoketal 7 . Here, the design of building block 7 , which contained a monoketal and a halogen atom X, contributed to the success of this strategy. The corresponding orthoquinone without the monoketal dimerizes as 4 (ref. 29 ). When X=H, a phenolic nucleophile causes an undesired C–C coupling [29] , presumably during competitive but reversible oxa-Michael addition. We expected the monoketal structure [34] and halogen X [35] , [36] , [37] , [38] to protect against self-dimerizations in 7 . The X also might enhance the elimination that occurred following oxa-Michael addition to make the addition irreversible. Moreover, the electronegativity of the halogen would limit the electrophilic position of oxa-Michael addition to the β-carbon of the aldehyde but not to that of the ketone. Transposition of the monoketal and ketone of 7 might increase steric hindrance and obstruct the approach of phenols. The coupled 12 required the reductive aromatization of the orthoquinone monoketal to obtain 13 . We achieved the selective reduction of the orthoquinone monoketal in the presence of an aldehyde, an ester in the ‘Aryl’ part, and a benzylidene acetal when 8 was used. Building block 7 resulted from oxidation of orthohalophenol 6 . Synthesis of the DHDG group As building block 7 , we prepared both bromide 7 -Br and iodide 7 -I ( Fig. 3 ). The preparation began with the successive benzylation of 8 and concurrent reduction of the methyl ester and regioselective cleavage of one C–O bond of the benzylidene group to give 15 . The regioselectivity resulted from the coordination of the reductant on the less sterically hindered outside oxygen of the benzylidene acetal. The aliphatic alcohol in 15 was oxidized by molecular oxygen under Uemura's conditions [39] to yield aldehyde 16 (ref. 40 ). No 16 was obtained through oxidations using MnO 2 , 2,2,6,6-tetramethylpiperidine 1-oxyl (TEMPO) and NaClO, TEMPO and (diacetoxyiodo)benzene, COCl 2 and dimethyl sulfoxide (DMSO), Dess-Martin periodinane, HBr and DMSO [41] , or HBr and H 2 O 2 (ref. 42 ). The bromination [43] , [44] and iodination of 16 provided 17 and 18 , respectively. Oxidation of phenols 17 and 18 with [bis(trifluoroacetoxy)iodo]benzene (PIFA) in the presence of benzyl alcohol [45] , [46] afforded orthoquinone monoketals 7 -Br and -I, both of which were stable and did not dimerize at room temperature. 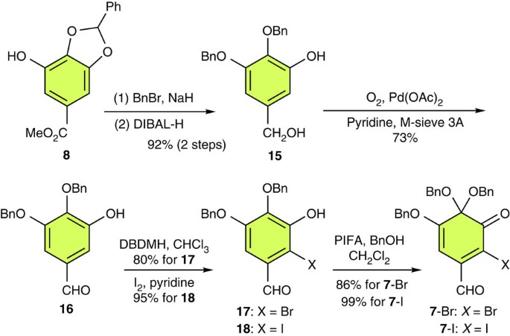Figure 3: Preparation of key building block 7. DBDMH, 1,3-dibromo-5,5-dimethylhydantoin; DIBAL-H, diisobutylaluminium hydride; Me, methyl; M-sieve, molecular sieves; PIFA, [bis(trifluoroacetoxy)iodo]benzene. Figure 3: Preparation of key building block 7. DBDMH, 1,3-dibromo-5,5-dimethylhydantoin; DIBAL-H, diisobutylaluminium hydride; Me, methyl; M-sieve, molecular sieves; PIFA, [bis(trifluoroacetoxy)iodo]benzene. Full size image Using building blocks 7 -Br and -I as electrophiles, we optimized the reaction conditions for oxa-Michael addition/elimination ( Fig. 4 ). Differently protected 8 and 9 were adopted as the nucleophiles. Among the four electrophile/nucleophile combinations, the reaction of 7 -Br with 8 was the fastest and gave the best yield. The reaction of 7 -I with 8 required a threefold longer reaction time (1.5 h) to finish and resulted in a slightly lower yield (89%). Thus, reactivity was opposite the performance of the leaving groups. The best combination, 7 -Br and 8 , consisted of the less sterically hindered electrophile and nucleophile; thus, the oxa-Michael addition might be the rate-limiting step of this sequence. The solvent effect was also remarkable. When the solvent (MeCN) was changed to DMSO, N,N -dimethylformamide (DMF), pyridine, EtOH, CH 2 Cl 2 , THF, or toluene, 19 was obtained in 99, 87, 59, 26, 0, 0, or 0% NMR yields, respectively, thereby demonstrating that the use of MeCN or DMSO is optimal. Adoption of other bases such as Na 2 CO 3 , Cs 2 CO 3 and K 3 PO 4 resulted in a lower yield under every combination of electrophile and nucleophile. 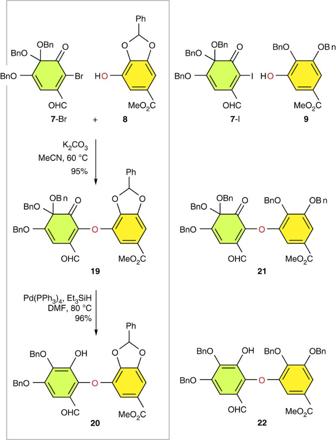Figure 4: Synthesis of the DHDG group. The first step is a subsequent oxa-Michael addition and elimination. Among all combinations with7-Br and7-I as the electrophiles and8and9as the nucleophiles, the combination of7-Br and8was the optimal one. The second step is a chemoselective reduction of the orthoquinone monoketal in the presence of the other reducible functional groups. The ketal and adjacent alkene acted as an allyl ether to form a Pd-π-allyl complex, which conferred chemoselectivity. DMF=N,N-dimethylformamide; Et, ethyl. Figure 4: Synthesis of the DHDG group. The first step is a subsequent oxa-Michael addition and elimination. Among all combinations with 7 -Br and 7 -I as the electrophiles and 8 and 9 as the nucleophiles, the combination of 7 -Br and 8 was the optimal one. The second step is a chemoselective reduction of the orthoquinone monoketal in the presence of the other reducible functional groups. The ketal and adjacent alkene acted as an allyl ether to form a Pd-π-allyl complex, which conferred chemoselectivity. DMF= N , N -dimethylformamide; Et, ethyl. Full size image We obtained the conditions for the chemoselective reduction of orthoquinone monoketal 19 ( Fig. 4 ) by considering the ketal and adjacent alkene as an allyl ether. This allyl ether could form its Pd-π-allyl complex and be reduced selectively [47] , [48] , [49] . Thus, treatment of 19 with catalytic Pd(PPh 3 ) 4 in the presence of Et 3 SiH in DMF gave 20 in 96% yield and demonstrated the development of a new synthetic method for the DHDG group. The solvent was selected after evaluation of MeCN, CH 2 Cl 2 , DMF, EtOH, THF and toluene. The optimal conditions were also applicable to 21 , yielding 22 in 95% yield. The results provided by other typical reductions were as follows. NaBH 4 reduced the aldehyde of 19 and thus did not provide the desired 20 , although simple orthoquinone monoketals are reduced by NaBH 4 (refs 50 , 51 ). The use of Et 3 SiH in the presence of TFA, which was a reduction condition of acetals [52] , produced a complex mixture. A radical reduction induced by n Bu 3 SnH and AIBN afforded 20 with a 51% yield, although such a radical reduction is uncommon for orthoquinone monoketals. Synthesis of the valoneoyl and tergalloyl groups We expanded the developed method to the valoneoyl and tergalloyl groups ( Fig. 5 ). For this purpose, phenols 24 and 31 were the nucleophiles to 7 -Br. Phenol 24 was prepared from known ( S )-HHDP compound 23 (ref. 53 ) via an eight-step protection/deprotection process ( Supplementary Methods 11–19 ). For the preparation of 31 , we developed C–C coupling of unequally protected gallates to avoid long protection/deprotection steps, similar to the preparation of 24 . Specifically, the intramolecular coupling of 28 ( Supplementary Methods 27–34 ), where the middle hydroxyl group of each galloyl group was protected by benzyl and 2-naphthylmethyl groups, was mediated by CuCl 2 – n BuNH 2 (ref 18 ) and afforded the corresponding coupled product 29 with an excellent yield. The subsequent methoxymethyl (MOM) protections for 30 and removal of the 2-naphthylmethyl group [54] gave 31 . The oxa-Michael addition/elimination of 24 and 31 with the building block 7 -Br furnished 25 and 32 , respectively. 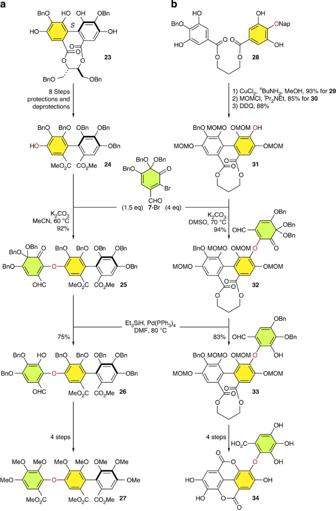Figure 5: Syntheses of the valoneoyl (a) and tergalloyl (b) groups. The sequence developed for the synthesis of the DHDG group—that is, oxa-Michael addition to7-Br, elimination and reductive aromatization—was applied to the synthesis of the valoneoyl and tergalloyl groups. These successful syntheses showed that the sequence was a unified method for the synthesis of C–O digallates. The intramolecular coupling of28is the first HHDP synthesis starting from unequally protected gallates. For structures of29and30, seeSupplementary Methods 35 and 36. Bu, butyl; DDQ, 2,3-dichloro-5,6-dicyano-p-benzoquinone; Nap, 2-naphthylmethyl; Pr, propyl. Figure 5: Syntheses of the valoneoyl ( a ) and tergalloyl ( b ) groups. The sequence developed for the synthesis of the DHDG group—that is, oxa-Michael addition to 7 -Br, elimination and reductive aromatization—was applied to the synthesis of the valoneoyl and tergalloyl groups. These successful syntheses showed that the sequence was a unified method for the synthesis of C–O digallates. The intramolecular coupling of 28 is the first HHDP synthesis starting from unequally protected gallates. For structures of 29 and 30 , see Supplementary Methods 35 and 36 . Bu, butyl; DDQ, 2,3-dichloro-5,6-dicyano- p- benzoquinone; Nap, 2-naphthylmethyl; Pr, propyl. Full size image To obtain excellent yields, the use of 1.5 and 4 equivalents of 7 -Br was required. Although 7 -Br was confirmed to be stable at 60 and 70 °C in MeCN and DMSO, respectively, for at least 10 h, the addition of K 2 CO 3 to each solution degraded 7 -Br. The degradation was faster in DMSO than in MeCN. Thus, in the degradation experiments, 7 -Br disappeared within 30 min at 70 °C in DMSO but 12% of 7 -Br was recovered after the reaction mixture was heated for 2 h in MeCN. However, when MeCN was used as the reaction solvent in the synthesis of 32 , the reaction rate decreased substantially. In the reactions that provided 25 and 32 , competition between the degradation of 7 -Br and the desired transformation required excess amounts of 7 -Br. The more obvious competition with 31 was due to increased steric hindrance around the nucleophilic oxygen atom. The chemoselective reduction of 25 and 32 provided 26 and 33 , respectively, whose structures contained the skeletons of valoneoyl and tergalloyl groups. These syntheses demonstrate the unified applicability of the method for the synthesis of C–O digallates. We confirmed the structures of 26 and 33 by transforming them to known compounds 27 (refs 25 , 55 ) ( Supplementary Tables 1 and 2 and Supplementary Methods 22–26 ) and 34 (ref. 56 ) ( Supplementary Table 3 and Supplementary Methods 40–43 ), respectively. Total synthesis of rugosin A The unified method paved the way for the total synthesis of rugosin A ( 2 , Fig. 1 ), an ellagitannin bearing a valoneoyl group. This ellagitannin was isolated from Rosa rugosa THUNB and characterized by Okuda et al . [57] The synthesis commenced with the preparation of 1,2,3-tri- O -galloylated β- D -glucose 36 ( Fig. 6 ). We prepared 36 from 4,6- O- benzylidene- D -glucose ( 35 ) [58] through galloylation of the triol followed by removal of the benzylidene group. Successive transformations—specifically, the double esterification [59] of 36 with 37 to provide the 4,6-( S )-HHDP bridged 38 , removal of the MOM groups for diol 39 and partial benzylation of free phenolic hydroxyl groups—yielded monohydroxy compound 40 along with its regioisomer 41 , a fully benzylated compound 42 (ref. 60 ), and recovered diol 39 . Separation of these four compounds was possible by silica-gel column chromatography eluted with a mixture of n- hexane, toluene and ethyl acetate (EtOAc). 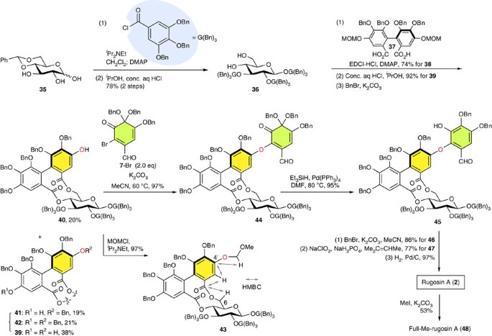Figure 6: Total synthesis of rugosin A (2). The unified method for the synthesis of C–O digallates was applied to the total synthesis of a natural ellagitannin. This example is the first total synthesis of a valoneoyl group containing ellagitannin. For structures of38,39,46and47, seeSupplementary Methods 46, 47, 53 and 54, respectively. aq, aqueous; conc., concentrated; DMAP, 4-(dimethylamino)pyridine; EDCI,N-(3-dimethylaminopropyl)-N′-ethylcarbodiimide; G(Bn)3, tri-O-benzylgalloyl; HMBC, heteronuclear multiple-bond correlation. We determined the position of the hydroxyl group in 40 as its MOM-protected form 43 by tracing heteronuclear multiple-bond correlation observed in THF- d 8 , as illustrated in Figure 6 . Each observation in acetone- d 6 , CDCl 3 and CD 3 CN gave inconclusive spectra due to overlapping of the critical peaks. The oxa-Michael addition/elimination with 40 and 7 -Br furnished the corresponding C–O-bonded orthoquinone monoketal 44 . Reduction of the orthoquinone monoketal produced 45 , which formed the skeleton of 2 . Finally, successive benzylation of the hydroxyl group of 45 to provide 46 , sodium chlorite-mediated oxidation [61] , [62] , [63] of the aldehyde to the corresponding carboxylic acid 47 , and complete debenzylation afforded 2 . The 1 H and 13 C NMR spectra of 2 were in agreement with those of the natural product; however, subtle differences in chemical shifts were observed ( Supplementary Tables 4 and 5 ). The identification of unprotected ellagitannins via NMR data is occasionally difficult because chemical shifts are prone to change due to the conditions of the observation. For example, the addition of D 2 O changed the proton nuclear magnetic resonance ( 1 H NMR) chemical shifts of 2 ( Fig. 7 ). Therefore, we identified the product after full methylation of synthesized 2 ; the 1 H NMR spectrum of fully methylated 48 was identical to that previously reported [57] ( Supplementary Table 6 ). Figure 6: Total synthesis of rugosin A (2). The unified method for the synthesis of C–O digallates was applied to the total synthesis of a natural ellagitannin. This example is the first total synthesis of a valoneoyl group containing ellagitannin. For structures of 38 , 39 , 46 and 47 , see Supplementary Methods 46, 47, 53 and 54 , respectively. aq, aqueous; conc., concentrated; DMAP, 4-(dimethylamino)pyridine; EDCI, N -(3-dimethylaminopropyl)- N ′-ethylcarbodiimide; G(Bn) 3 , tri- O -benzylgalloyl; HMBC, heteronuclear multiple-bond correlation. 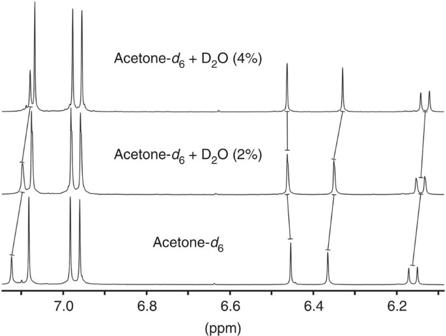Figure 7: Variable1H NMR chemical shift of 2. The chemical shifts in the1H NMR spectra changed after the addition of D2O to a solution of2in acetone-d6. This behaviour did not allow the complete identification of synthesized2by comparison with the1H NMR spectrum of natural2. Therefore, we prepared the permethylated analogue48(Fig. 6) for identification. Full size image Figure 7: Variable 1 H NMR chemical shift of 2. The chemical shifts in the 1 H NMR spectra changed after the addition of D 2 O to a solution of 2 in acetone- d 6 . This behaviour did not allow the complete identification of synthesized 2 by comparison with the 1 H NMR spectrum of natural 2 . Therefore, we prepared the permethylated analogue 48 ( Fig. 6 ) for identification. Full size image The creation of building block 7 -Br made possible a unified synthetic approach to C–O digallates with DHDG, valoneoyl and tergalloyl groups. This method features the oxa-Michael addition of a phenolic nucleophile to 7 -Br, subsequent elimination and reduction of the orthoquinone monoketal. In addition, we report the following three new achievements: (1) the syntheses of the valoneoyl and tergalloyl groups into a form that could be applicable for the total synthesis of unprotected ellagitannins, (2) the improvement in the method of synthesizing the HHDP group through intramolecular aryl–aryl coupling between unequally protected gallates, and (3) the total synthesis of the valoneoyl-group-containing ellagitannin. Because C–O digallates have frequently appeared in natural ellagitannins as key constituents to induce structural diversity, this work increases the number of synthetically available ellagitannins in an innovative manner. General Reactions were performed under an N 2 or Ar atmosphere unless otherwise noted. The phrase ‘the general drying procedure’ indicates successive treatments consisting of MgSO 4 -drying of an organic layer after extraction, removal of MgSO 4 by filtration and concentration of the filtrate. For detailed general methods, compound characterization data, and 1 H and 13 C NMR spectra of the compounds prepared in this study, see Supplementary Method 1, 2–54 and Supplementary Figs 1–51 , respectively. Synthesis of compound 15 A mixture of 8 (ref. 32 ) (1.00 g, 3.67 mmol), NaH (60% in mineral oil 220 mg, 132 mg as NaH, 5.51 mmol) and BnBr (942 mg, 5.51 mmol) in DMF and toluene (v/v=3/1, 37 ml) was stirred for 2 h at room temperature (RT). After the addition of satd aq NH 4 Cl (20 ml), the aq mixture was extracted with Et 2 O. The organic layer was successively washed with H 2 O and brine. After the general drying procedure, the resulting residue was purified by column chromatography (CC) (30 g of SiO 2 , n- hexane/EtOAc=20/1 to 5/1) to afford the corresponding benzyl ether (1.22 g, 92% yield) as a white solid. Diisobutylaluminium hydride (1.0 M in THF, 9.7 ml, 9.7 mmol) was added to a solution of the benzyl ether (1.00 g, 2.78 mmol) in CH 2 Cl 2 (10 ml). The solution was stirred for 1 h at 0 °C. After the addition of 1 M hydrochloric acid (20 ml), the aq mixture was extracted with EtOAc. The organic layer was successively washed with 1 M hydrochloric acid, H 2 O and brine. After the general drying procedure, the resulting residue was purified by CC (20 g of SiO 2 , n -hexane/EtOAc=5/1 to 1/1) to afford 15 (935 mg, 100% yield) as a colourless syrup. Synthesis of compound 16 A mixture of 15 (220 mg, 654 μmol), pyridine (51.7 mg, 654 μmol), activated 3 A molecular sieves (300 mg) and Pd(OAc) 2 (14.7 mg, 65.4 μmol) in DMF (6.5 ml) was stirred for 18 h at 90 °C under an O 2 atmosphere. After the addition of Et 2 O (5 ml) and 1 M hydrochloric acid (15 ml), the aq mixture was extracted with Et 2 O. The organic layer was washed with satd aq NaHCO 3 . After the general drying procedure, the resulting residue was purified by CC (7.0 g of SiO 2 , n- hexane/EtOAc=15/1 to 4/1) to afford 16 (159 mg, 73% yield) as a white solid. 1 H NMR data for 16 were identical to those previously reported [40] . Synthesis of compound 17 A mixture of 1,3-dibromo-5,5-dimethylhydantoin (428 mg, 1.50 mmol) and 16 (1.00 g , 2.99 mmol) in CHCl 3 (30 ml) was stirred for 24 h at RT. After the addition of 10% aq Na 2 S 2 O 3 , the aq mixture was extracted with Et 2 O. The organic layer was washed with H 2 O. After the general drying procedure, the crude product was purified by crystallization (EtOAc/ n -hexane) to afford 17 (994 mg, 80% yield) as a white solid. Synthesis of compound 18 A mixture of 16 (50.0 mg, 150 μmol), pyridine (29.1 mg, 369 μmol) and I 2 (45.5 mg, 179 μmol) in CHCl 3 (1.5 ml) was stirred for 4 h at RT. Further I 2 (23.9 mg, 94.2 μmol) was added, and the mixture was stirred for an additional 20 h. After 10% aq Na 2 S 2 O 3 was added until the mixture became colourless (5 ml), the aq mixture was extracted with Et 2 O. The organic layer was successively washed with H 2 O, 1 M hydrochloric acid and brine. After the general drying procedure, the resulting residue was purified by CC (3 g of SiO 2 , n -hexane/EtOAc=15/1 to 7/1) to afford 18 (65.6 mg, 95% yield) as a white solid. Synthesis of compound 7-Br PIFA (563 mg, 1.31 mmol) was added to a solution of 17 (360 mg, 872 μmol) in CH 2 Cl 2 (2.0 ml) and BnOH (3.0 ml). The solution was stirred for 5 min at RT. After the addition of Et 2 O (30 ml) and satd aq NaHCO 3 (10 ml), the aq mixture was extracted with Et 2 O. The organic layer was successively washed with H 2 O. After the general drying procedure, the resulting residue was purified by CC (90 g of SiO 2 , n -hexane/toluene=1/0 to 1/2 to 1/3) to afford 7 -Br (390 mg, 86% yield) as a red syrup. Synthesis of compound 7-I A mixture of 18 (300 mg, 652 μmol) and PIFA (336 mg, 782 μmol) in CH 2 Cl 2 (1.0 ml) and BnOH (5.0 ml) was stirred for 5 min at RT. After the addition of Et 2 O (20 ml) and satd aq NaHCO 3 (10 ml), the aq mixture was extracted with Et 2 O. The organic layer was washed with H 2 O. After the general drying procedure, the resulting residue was purified by CC (9.0 g of SiO 2 , n -hexane/EtOAc=50/1 to 15/1) to afford 7 -I (366 mg, 99% yield) as a red syrup. Reaction of 7-Br with 8 A mixture of 7 -Br (53.4 mg, 103 μmol), 8 (36.5 mg, 134 μmol) and K 2 CO 3 (71.2 mg, 515 μmol) in MeCN (1.4 ml) was stirred for 30 min at 60 °C. After the mixture was cooled to RT, Et 2 O (5 ml) and 1 M hydrochloric acid (5 ml) were added. The aq mixture was extracted with Et 2 O. The organic layer was successively washed with satd aq NaHCO 3 and brine. After the general drying procedure, the crude product was purified by CC (2.0 g of SiO 2 , n- hexane/EtOAc=20/1 to 10/1) to afford 19 (69.3 mg, 95% yield) as a red syrup. Reaction of 7-I with 8 In a reaction similar to that described in the previous procedure, the use of 7 -I (43.0 mg, 75.9 μmol), 8 (26.9 mg, 98.7 μmol) and K 2 CO 3 (40.9 mg, 296 μmol) provided a crude product containing 19 . The reaction time was 1.5 h. The crude product was purified by CC (2.0 g of SiO 2 , n- hexane/EtOAc=20/1 to 6/1) to afford 19 (48.1 mg, 89% yield). Reaction of 7-Br with 9 In a reaction similar to that described for 7 -Br and 8 , the use of 7 -Br (20.3 mg, 39.1 μmol), 9 (18.9 mg, 50.8 μmol) and K 2 CO 3 (27.0 mg, 195 μmol) provided 21 (18.9 mg, 60% yield) as a red syrup. The reaction time was 50 min. Reaction of 7-I with 9 In a reaction similar to that described for 7 -Br and 8 , the use of 7 -I (10.0 mg, 17.7 μmol), 9 (8.4 mg, 22.9 μmol), K 2 CO 3 (12.3 mg, 89.3 μmol) and MeCN (1.0 ml) provided a crude product containing 21 . The yield of 21 was 46% on the basis of the 1 H NMR spectra of the crude product. Synthesis of compound 20 Pd(PPh 3 ) 4 (4.8 mg, 4.2 μmol) was added to a solution of 19 (59.6 mg, 83.9 μmol) and Et 3 SiH (19.5 mg, 168 μmol) in DMF (1.0 ml). The solution was stirred for 15 min at 80 °C. After the mixture cooled to RT, Et 2 O (5 ml) and 1 M hydrochloric acid (5 ml) were added. The aq mixture was extracted with Et 2 O. The organic layer was successively washed with satd aq NaHCO 3 and brine. After the general drying procedure, the crude product was purified by CC (1.0 g of SiO 2 , n- hexane/EtOAc=20/1 to 5/1) to afford 20 (48.8 mg, 96%) as a pale yellow syrup. Synthesis of compound 22 In a reaction similar to that described for the synthesis of 20 , the use of 21 (52.0 mg, 64.8 μmol), Et 3 SiH (15.1 mg, 130 μmol) and Pd(PPh 3 ) 4 (0.7 mg, 0.6 μmol) provided 22 (42.8 mg, 95% yield) as a colourless syrup after purification by CC (1.0 g of SiO 2 , n -hexane/EtOAc=10/1 to 5/1). Synthesis of compound 25 A mixture of 7 -Br (81.6 mg, 157 μmol), 24 (85.6 mg, 105 μmol) and K 2 CO 3 (72.6 mg, 525 μmol) in MeCN (1.0 ml) was stirred for 2 h at 60 °C. After the addition of Et 2 O (5.0 ml) and 1 M hydrochloric acid (5.0 ml), the aq mixture was extracted with Et 2 O. The organic layer was successively washed with satd aq NaHCO 3 and brine. After the general drying procedure, the crude product was purified by CC (8.0 g of SiO 2 , n -hexane/EtOAc=10/1 to 3/1) to afford 25 (121 mg, 92% yield) as a red syrup. Synthesis of compound 26 A mixture of 25 (244 mg, 194 μmol), Et 3 SiH (33.8 mg, 291 μmol) and Pd(PPh 3 ) 4 (22.4 mg, 19.4 μmol) in DMF (2.0 ml) was stirred for 10 min at 80 °C. After the addition of Et 2 O (3.0 ml) and H 2 O (3.0 ml), the aq mixture was extracted with Et 2 O. The organic layer was successively washed with satd aq NaHCO 3 and brine. After the general drying procedure, the crude product was purified by CC (8.0 g of SiO 2 , n -hexane/EtOAc=10/1 to 3/1) to afford 26 (168 mg, 75% yield) as a colourless syrup. Synthesis of compound 32 A mixture of 7 -Br (268 mg, 516 μmol), 31 (83.0 mg, 129 μmol) and K 2 CO 3 (89.1 mg, 645 μmol) in DMSO (1.3 ml) was stirred for 15 min at 70 °C. After the addition of Et 2 O (5 ml) and 1 M hydrochloric acid (5 ml), the aq mixture was extracted with Et 2 O. The organic layer was successively washed with satd aq NaHCO 3 and brine. After the general drying procedure, the resulting residue was purified by CC (2.5 g of SiO 2 , n -hexane/toluene/Et 2 O=5/3/2 to 2/3/2) to afford 32 (131 mg, 94% yield) as a red syrup. Synthesis of compound 33 A mixture of 32 (80.5 mg, 74.3 μmol), Et 3 SiH (13.0 mg, 111 μmol) and Pd(PPh 3 ) 4 (8.6 mg, 7.4 μmol) in DMF (6.0 ml) was stirred for 10 min at 80 °C. After the addition of Et 2 O (3 ml) and 1 M hydrochloric acid (3 ml), the aq mixture was extracted with Et 2 O. The organic layer was successively washed with satd aq NaHCO 3 and brine. After the general drying procedure, the resulting residue was purified by CC (2.5 g of SiO 2 , n -hexane/toluene/EtOAc=5/3/1 to 2/3/2) to afford 33 (60.1 mg, 83% yield) as a colourless syrup. Synthesis of compound 36 A mixture of 3,4,5-tri- O -benzylgallic acid [64] (821 mg, 1.86 mmol), oxalyl chloride (360 mg, 2.84 mmol) and DMF (0.1 ml) in toluene (10 ml) was stirred for 45 min at 70 °C. The reaction mixture was concentrated, and toluene (10 ml) was added to the residue. The desired acid chloride dissolved into toluene, whereas a yellow and highly viscous side-product remained undissolved. Thus, the toluene solution was decanted into another flask, and the former flask was rinsed with toluene (5 ml). The combined toluene solution was concentrated to afford 3,4,5-tri- O -benzylgallic acid chloride as a yellow syrup. Without purification, the crude product was used in the next reaction. To a solution of 35 (ref. 58 ) (100 mg, 373 μmol) and i Pr 2 NEt (1.5 ml) in CH 2 Cl 2 (10 ml) was added a solution of the acid chloride in CH 2 Cl 2 (10 ml). After the mixture was stirred for 25 h at RT, 4-(dimethylamino)pyridine (2.1 mg, 17.2 μmol) was added. The mixture was stirred for 24 h at reflux. After the addition of MeOH (5 ml) and H 2 O (10 ml), the aq mixture was extracted with EtOAc. The organic layer was successively washed with H 2 O and brine. After the general drying procedure, a mixture of desired trigallate and 3,4,5-tri- O -benzylgallic anhydride was obtained through crystallization (benzene/ n -hexane), which was used for the next transformation. To a solution of the product (672 mg) in THF (8.0 ml) was added a mixture of i PrOH and conc. hydrochloric acid (v/v=50/1, 4.0 ml). After being stirred for 22 h at 55 °C, the mixture was concentrated to remove the i PrOH and THF. The remaining aq mixture was extracted with Et 2 O. The organic layer was successively washed with satd aq NaHCO 3 and brine. After the general drying procedure, the resulting residue was purified by CC (30 g of SiO 2 , n -hexane/EtOAc=2/1 to 1/1.5) to afford 36 (416 mg, 78% yield from 35 ) as a colourless amorphous solid. Synthesis of compound 38 A mixture of 36 (350 mg, 241 μmol), 37 (228 mg, 290 μmol), 4-(dimethylamino)pyridine (36 mg, 290 μmol) and N -(3-dimethylaminopropyl)- N' -ethylcarbodiimide·HCl (111 mg, 578 μmol) in CH 2 Cl 2 (24 ml) was stirred for 3 h at 0 °C followed by for 18 h at RT. After the addition of EtOAc (20 ml) and 1 M hydrochloric acid (20 ml), the aq mixture was extracted with EtOAc. The organic layer was successively washed with H 2 O and brine. After the general drying procedure, the crude product was purified by CC (15 g of SiO 2 , n -hexane/EtOAc=5/1 to 2/1) to afford 38 (393 mg, 74% yield) as a colourless amorphous solid. Synthesis of compound 39 To a solution of 38 (163 mg, 74.1 μmol) in THF (3.0 ml) was added a mixture of i PrOH and conc. hydrochloric acid (v/v=50/1, 1.0 ml). The mixture was stirred for 26 h at 55 °C. After the addition of satd aq NaHCO 3 (10 ml), the mixture was extracted with Et 2 O. The organic layer was successively washed with H 2 O and brine. After the general drying procedure, the crude product was purified by CC (5 g of SiO 2 , n -hexane/EtOAc=5/1 to 2/1) to afford 39 (144 mg, 92%) as a colourless syrup. Synthesis of compound 40 A mixture of 39 (454 mg, 215 μmol), K 2 CO 3 (323 mg, 2.34 mmol) and BnBr (36.8 mg, 215 μmol) in DMF (2.5 ml) was stirred for 5.5 h at RT. After the addition of Et 2 O (5.0 ml) and 1 M hydrochloric acid (5.0 ml), the aq mixture was extracted with Et 2 O. The organic layer was successively washed with satd aq NaHCO 3 and brine. After the general drying procedure, the crude product was purified by CC (50 g of SiO 2 , n -hexane/toluene/EtOAc=20/5/2 to 5/5/2) to afford 40 (76.8 mg, 20% yield) as a colourless syrup, 41 (71.4 mg, 19%) as a colourless syrup, full-Bn tellimagrandin II ( 42 ) (83.0 mg, 21%) as a colourless amorphous solid, and recovered 39 (132 mg, 38%). The 1 H NMR data of 42 were identical to those previously reported [60] . Synthesis of compound 43 A mixture of 40 (15.6 mg, 7.09 μmol), i Pr 2 NEt (2.3 mg, 18 μmol) and MOMCl (0.9 mg, 10 μmol) in CH 2 Cl 2 (0.5 ml) was stirred for 1 h at RT. After the addition of Et 2 O (5 ml) and 1 M hydrochloric acid (3 ml), the aq mixture was extracted with Et 2 O. The organic layer was successively washed with H 2 O and brine. After the general drying procedure, the crude product was purified by CC (1.0 g of SiO 2 , n -hexane/EtOAc=5/1 to 2/1) to afford 43 (15.5 mg, 97% yield) as a colourless syrup. Synthesis of compound 44 A solution of 7 -Br (88.8 mg, 171 μmol), 40 (188 mg, 85.4 μmol) and K 2 CO 3 (59.0 mg, 427 μmol) in MeCN (1.0 ml) was stirred for 2 h at 60 °C. After the addition of Et 2 O (5.0 ml) and 1 M hydrochloric acid (5.0 ml), the aq mixture was extracted with Et 2 O. The organic layer was successively washed with satd aq NaHCO 3 and brine. After the general drying procedure, the crude product was purified by CC (6.0 g of SiO 2 , n -hexane/EtOAc=10/1 to 2/1) to afford 44 (218 mg, 97% yield) as a red syrup. Synthesis of compound 45 A mixture of 44 (332 mg, 126 μmol), Et 3 SiH (22.0 mg, 189 μmol) and Pd(PPh 3 ) 4 (14.6 mg, 12.6 μmol) in DMF (1.5 ml) was stirred for 10 min at 80 °C. After the addition of Et 2 O (3.0 ml) and H 2 O (3.0 ml), the aq mixture was extracted with Et 2 O. The organic layer was successively washed with satd aq NaHCO 3 and brine. After the general drying procedure, the crude product was purified by CC (10 g of SiO 2 , n -hexane/toluene/EtOAc=30/5/2 to 8/5/2) to afford 45 (306 mg, 95% yield) as a pale yellow syrup. Synthesis of compound 46 A mixture of 45 (306 mg, 102 μmol), K 2 CO 3 (70.5 mg, 510 μmol) and BnBr (26.2 mg, 153 μmol) in MeCN (1.5 ml) was stirred for 8.5 h at RT. After the addition of Et 2 O (5.0 ml) and 1 M hydrochloric acid (5.0 ml), the aq mixture was extracted with Et 2 O. The organic layer was successively washed with satd aq NaHCO 3 and brine. After the general drying procedure, the crude product was purified by CC (15 g of SiO 2 , n -hexane/toluene/EtOAc=30/5/2 to 12/5/2) to afford 46 (230.8 mg, 86% yield) as a colourless syrup. Synthesis of compound 47 To a stirred solution of 46 (238 mg, 88.0 μmol), 2-methyl-2-butene (0.1 ml) and NaH 2 PO 4 (20.6 mg, 132 μmol) in THF/ t BuOH (v/v=1/1, 2.0 ml) was added a solution of NaClO 2 (11.9 mg, 132 μmol) in H 2 O (0.5 ml). The reaction mixture was stirred at RT for 30 min under air. After the addition of H 2 O (5.0 ml), the aq mixture was extracted with Et 2 O. The organic layer was successively washed with satd aq NaHCO 3 and brine. After the general drying procedure, the resulting residue was purified by CC (5.0 g of SiO 2 , n -hexane/toluene/EtOAc=10/5/2 to 5/0/1 to 1/0/1) to afford 47 (179 mg, 77% yield) as a pale yellow syrup. Synthesis of compound 2 A mixture of 47 (22.5 mg, 8.53 μmol) and Pd on carbon (10 wt.%, 5.0 mg) in acetone (1.0 ml) was stirred for 5.5 h at RT under a H 2 atmosphere. The mixture was filtered through a cotton–Celite pad to remove the catalyst and carbon. The crude product was dissolved in 1 M hydrochloric acid and purified by CC (500 mg of Sephadex LH-20, H 2 O to MeOH) to afford 2 (9.2 mg, 97% yield) as a pale yellow syrup. 1 H NMR, 13 C NMR, HRMS and optical rotation data for 2 were in agreement with those previously reported [57] . Synthesis of compound 48 A mixture of synthesized 2 (5.5 mg, 4.97 μmol), K 2 CO 3 (65.0 mg, 470 μmol) and MeI (228 mg, 1.61 μmol) in DMF (0.25 ml) was stirred for 10 min at RT. After the addition of 1 M hydrochloric acid (3.0 ml), the aq mixture was extracted with Et 2 O. The organic layer was successively washed with satd aq NaHCO 3 and brine. After the general drying procedure, the resulting residue was purified by CC (500 mg of SiO 2 , n- hexane/EtOAc=5/1 to 1/2) to afford 48 (3.6 mg, 53% yield) as a pale yellow syrup. 1 H NMR and optical rotation data for 48 were identical to those previously reported [57] . How to cite this article : Hirokane, T. et al. A unified strategy for the synthesis of highly oxygenated diaryl ethers featured in ellagitannins. Nat. Commun. 5:3478 doi: 10.1038/ncomms4478 (2014).